High lithium anodic performance of highly nitrogen-doped porous carbon prepared from a metal-organic framework Theoretical and experimental results have revealed that the lithium-ion storage capacity for nitrogen-doped graphene largely depends on the nitrogen-doping level. However, most nitrogen-doped carbon materials used for lithium-ion batteries are reported to have a nitrogen content of approximately 10 wt% because a higher number of nitrogen atoms in the two-dimensional honeycomb lattice can result in structural instability. Here we report nitrogen-doped graphene particle analogues with a nitrogen content of up to 17.72 wt% that are prepared by the pyrolysis of a nitrogen-containing zeolitic imidazolate framework at 800 °C under a nitrogen atmosphere. As an anode material for lithium-ion batteries, these particles retain a capacity of 2,132 mA h g −1 after 50 cycles at a current density of 100 mA g −1 , and 785 mAh g −1 after 1,000 cycles at 5 A g −1 . The remarkable performance results from the graphene analogous particles doped with nitrogen within the hexagonal lattice and edges. Lithium-ion batteries (LIBs) with high storage capacities and excellent rate performance have been widely considered as a promising power source for portable electronic devices [1] , [2] , [3] , [4] . Graphite, the commercial anode material, cannot meet the increasing demands of rapidly developing LIB markets due to its low theoretical specific capacity (372 mA h g −1 ) [5] . In recent years, various nanostructured Si (ref. 6 ), Sn (ref. 7 ), SnO 2 (ref. 8 ) and some transition metal oxides [9] , [10] with ultra-high theoretical capacities have been explored as anode materials for LIBs due to their special mechanisms for Li storage. Unfortunately, the large voltage hysteresis (in conventional electrodes) and huge volume expansion (in alloying electrodes) that occur in these materials during the Li insertion and extraction process severely limit their extensive applications in LIBs [11] , [12] . Therefore, researchers have continuously focused on preparing novel carbon-based anode materials with enhanced electrochemical performances for Li storage by virtue of their excellent cycling stability and high electrical conductivity. To date, several novel carbon-based anode materials with various structures have been extensively investigated for applications in LIBs, such as carbon nanotubes (625 mA h g −1 ) (ref. 13 ), graphene (approximately 568 mA h g −1 ) (ref. 14 ) and carbon nanotube and graphene composites [15] , [16] . In addition, partially graphitized porous carbon is a class of emerging materials with promising chemical properties for LIBs due to their relatively low cost, high conductivity and porous structure, which make them very attractive materials. For example, Zhang and co-workers [17] reported the template-free synthesis of hollow carbon nanospheres for high-performance anode materials for LIBs (630 mA h g −1 after 50 cycles). In addition, the chemical and electronic properties of the carbon hosts can be further modified by doping with heteroatoms, such as phosphorus [18] , boron [19] , sulfur [20] and nitrogen [21] . The heteroatom-doped carbon materials have substantially greater specific capacities and excellent cycling stability relative to non-doped carbon materials. Of these various heteroatom-doped carbon materials, nitrogen-doped (N-doped) carbon materials are attractive because their electronegativity (3.5) is higher than that of carbon (3.0) and their atomic diameter is smaller [22] . Moreover, the N atoms incorporated into graphitic networks facilitate the formation of stronger interactions between the N-doped carbon structure and the Li ions, which are favourable for Li insertion. For example, Wang et al . [23] reported that doping with 3.9 atom% nitrogen could improve the Li storage capacity by up to 600 mAh g −1 , which is higher than pure graphene. Wang et al . [22] reported that N-doped graphene nanosheets exhibit a high reversible capacity of up to 900 mA h g −1 and a significantly enhanced cycling stability. In addition, theoretical calculations showed that the N-doped graphene with all N atoms doped within its lattice exhibits superior electrochemical performance with a capacity of up to 1,262 mA h g −1 (ref. 24 ). However, most of the reported N-doped carbon materials for LIBs have a N content of approximately 10 wt% (ref. 25 ). Theoretical calculations have shown that a large quantity of N atoms in the two-dimensional (2D) graphene lattice can result in structural instability [26] . Carbon matrixes, especially those obtained through solution methods, contain large amounts of hydroxyl, epoxy, carbonyl and carboxyl groups, which usually occupy the active sites on their surfaces and edges, resulting in less active sites for grafting N atoms. Therefore, the fabrication of carbon materials without oxygen-bearing groups could be an efficient method for increasing the N content of carbon materials, which could provide more active sites at their edges for grafting N atoms, especially pyridinic N and pyrrolic N. Metal-organic frameworks (MOFs) generated from a supramolecular assembly of inorganic components (metal ions or metal clusters) with organic components (organic or organometallic complexes) represent an emerging class of materials that have attracted extensive research interest because of their versatile functionalities and tunable porosities [27] . Due to their permanent nanoscale cavities and open channels, which are similar to mesoporous silicas and zeolites, MOFs exhibit a strong potential for use as templates and reactive precursors for synthesizing nanoporous carbon materials [28] , [29] . In addition, research has continuously focused on preparing metal oxides through the direct calcination of various MOFs [30] , [31] , [32] . However, no attention has been given to the creation of high-level heteroatom-doped carbon materials through direct pyrolysis of MOFs, which contain heteroatoms in their organic components, such as phosphorus, boron, sulfur and nitrogen [33] , [34] , [35] . In addition, direct pyrolysis of MOFs may be an efficient method for avoiding the generation of oxygen-bearing groups, such as hydroxyl groups, in the resulting carbon materials. Thus, it is highly desirable to produce small graphene particle analogues via the direct carbonation of N-containing MOFs in an inert atmosphere to achieve high-level N doping. The ZIF-8 framework consists of the Zn 2+ transition metal ion and N-containing 2-methylimidazolate linkers (34 wt% N), which can form three-dimensional (3D) frameworks resembling zeolite topologies [36] . Here we design a facile strategy for fabricating high-level N-doped microporous carbon polyhedrons by the pyrolysis of ZIF-8 polyhedrons. The resulting product inherits the structural characteristics of the parent ZIF-8 particles and can be considered as an aggregate of large amounts of small graphene analogous particles, which can provide abundant active sites on their surfaces and at their edges for grafting nitrogen atoms. The high-level N-doped graphene analogous particles exhibit excellent electrochemical performance as an anode material for LIBs. This remarkable electrochemical performance can be attributed to the unique N-doped carbon structure, which consists of large amounts of small graphene analogous particles that are highly doped with N within the hexagonal lattice and edges. Characterization A facile two-step strategy, which includes the large-scale fabrication of N-containing ZIF-8 precursors at room temperature and subsequent thermal annealing under a N 2 atmosphere for carbonization, was developed to prepare high-level N-doped graphene analogous particles. Briefly, the N-containing ZIF-8 precursor was synthesized by reacting 2-methylimidazole with Zn(NO 3 ) 2 in methanol at room temperature for 10 h. Herein, the ZIF-8 framework [Zn(MeIM) 2 ; MeIM=2-methylimidazole], including 2-methylimidazole (34 wt% N), acts as a sacrificial template and precursor to prepare the aggregates of the N-doped graphene analogous particles without adding any carbon sources, such as glucose and sucrose. In addition, the resulting sample inherits the shape of the ZIF-8 particles and has a high N content (17.72 wt%). 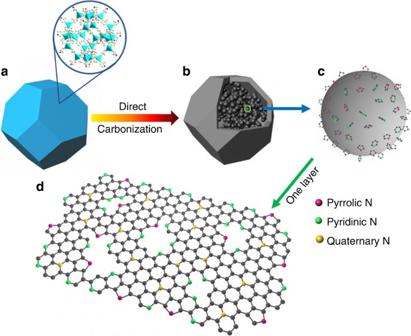Figure 1: Schematic illustration of the synthesis procedure of N-doped graphene analogous particles and model of N-doping. (a) ZIF-8. (b) N-rich carbon polyhedron containing large amounts of graphene analogous particles. (c) Enlargement of one graphene particle analogues, which contains several graphene layers and can provide abundant active sites at their edges for grafting nitrogen heteroatoms. (d) The schematic of three types of bonding configurations of N atoms within the hexagonal lattice and edges of a graphene layer. Figure 1 shows the entire synthetic route and structure of the N-doped graphene analogous particles. Figure 1: Schematic illustration of the synthesis procedure of N-doped graphene analogous particles and model of N-doping. ( a ) ZIF-8. ( b ) N-rich carbon polyhedron containing large amounts of graphene analogous particles. ( c ) Enlargement of one graphene particle analogues, which contains several graphene layers and can provide abundant active sites at their edges for grafting nitrogen heteroatoms. ( d ) The schematic of three types of bonding configurations of N atoms within the hexagonal lattice and edges of a graphene layer. Full size image The product exhibits a polyhedron-like morphology with a diameter of approximately 200 nm ( Supplementary Fig. 1a,b ). The transmission electron microscopy (TEM) analysis results ( Supplementary Fig. 1c,d ) are consistent with the field emission scanning electron microscopy (FESEM) results. The X-ray diffraction (XRD) pattern of the as-prepared ZIF-8 precursor is identical to its corresponding simulated pattern, as shown by its crystallographic data ( Supplementary Fig. 2a ). From the thermogravimetric analysis (TGA) results ( Supplementary Note 1 ), it was concluded that the 3D ZIF-8 framework possesses the highest thermal stability. This high thermal stability is advantageous for a carbonization precursor because high-temperature vaporization can be avoided. On the basis of the TGA–infrared (IR)–mass spectrometry (MS) results ( Supplementary Fig. 3 ; Supplementary Note 2 ), NH 3 and (CN) 2 molecules were produced during the carbonation process. Interestingly, when the carbonation temperature was increased to 700 °C, gaseous molecules were not produced. The optical micrographs of the precursor and the prepared samples are shown in Supplementary Fig. 4 . The XRD patterns of the N-doped graphene analogous particles (N-C-600, N-C-700, N-C-800 and N-C-900) are shown in Fig. 2a and in Supplementary Figs 5–7 . These particles exhibited similar diffraction features with a broad peak at approximately 2 θ =24°, corresponding to the carbon (002) peak that is typical of graphitic carbon materials with a low degree of graphilization [37] . No other impurities, such as ZnO or Zn, were observed in the XRD patterns. 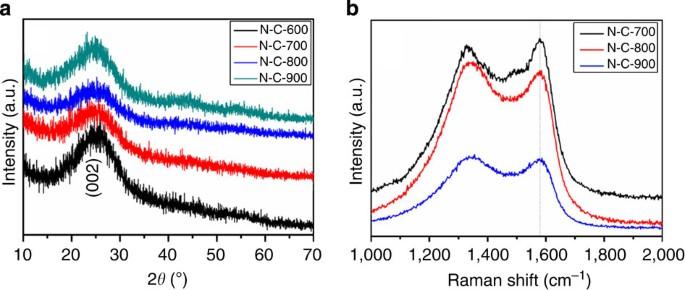Figure 2: Structural evolution of N-doped graphene analogous particles by XRD and Raman spectroscopy. (a) XRD patterns and (b) Raman spectra of N-doped graphene analogous particles obtained at different calcination temperatures. Figure 2b and Supplementary Fig. 8 show the Raman spectra for the obtained N-doped graphene analogous particles. The G band is a characteristic feature of graphitic layers, while the D band corresponds to disordered carbon or defective graphitic structures. Raman spectroscopy is sensitive to subtle structural variations in carbon materials. A high I D /I G band intensity ratio indicates the generation of large amounts of defects [38] , [39] , [40] , which suggests that the edge modification of N atoms in graphene analogous particles occurred in our samples. The I D /I G ratio for C-N-800 is greater than that of C-N-700 and C-N-900, demonstrating more N-doping atoms at the edges of the N-doped graphene analogous particles. In addition, a broad and weak second-order band was observed at approximately 2,700 cm −1 for N-C-800 ( Supplementary Fig. 9 ) and the shape of the D and 2D bands (more specifically the absence of a typical graphite shoulder) are characteristic features of few-layered graphene [24] , [39] , [40] . Figure 2: Structural evolution of N-doped graphene analogous particles by XRD and Raman spectroscopy. ( a ) XRD patterns and ( b ) Raman spectra of N-doped graphene analogous particles obtained at different calcination temperatures. Full size image As observed by FESEM and TEM ( Fig. 3a,b ), the as-synthesized N-C-800 inherited the original morphology of the ZIF-8 particles, even after high-temperature thermal treatment under a N 2 atmosphere. However, the surfaces of the carbon samples became rough after carbonization and washing with an aqueous HCl solution. The selected-area electron diffraction pattern ( Fig. 3c ) displays a typical ring feature, which indicates an amorphous character. The high-resolution transmission electron microscope (HRTEM) image ( Fig. 3d ) at the edge of the polyhedron clearly shows the presence of oriented multilayer domains and several graphene layers stacked in parallel with an adjacent interlayer distance of approximately 0.34 nm. This observation is consistent with the d-spacing of the (002) crystal plane of bulk graphite. As shown in Fig. 3 , the images of elemental mapping by energy-filtered TEM (EFTEM) reveal that a large quantity of N atoms are effectively incorporated into the skeletons of the N-C-800 polyhedrons. Furthermore, electron energy loss spectroscopy revealed the simultaneous presence of C and N in the N-C-800 ( Supplementary Fig. 10 ). The samples prepared at other temperatures had similar morphologies and microstructures to those of N-C-800 ( Supplementary Fig. 11 ). 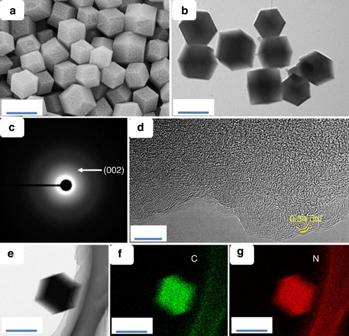Figure 3: Structural evolution of N-doped graphene analogous particles by electron microscopy. (a) FESEM and (b) TEM images of the MOF-derived mesoporous N-C-800 polyhedrons. (c) Selected-area electron diffraction pattern of the MOF-derived mesoporous N-C-800 polyhedrons. (d) HRTEM image of the MOF-derived mesoporous N-C-800 polyhedrons. (e–g) Scanning TEM image of the MOF-derived mesoporous N-C-800 polyhedron and energy dispersive X-ray spectrometry elemental maps of C and N, repectively. Scale bars;a,b(200 nm);d(5 nm);e,f,g(200 nm). Figure 3: Structural evolution of N-doped graphene analogous particles by electron microscopy. ( a ) FESEM and ( b ) TEM images of the MOF-derived mesoporous N-C-800 polyhedrons. ( c ) Selected-area electron diffraction pattern of the MOF-derived mesoporous N-C-800 polyhedrons. ( d ) HRTEM image of the MOF-derived mesoporous N-C-800 polyhedrons. ( e – g ) Scanning TEM image of the MOF-derived mesoporous N-C-800 polyhedron and energy dispersive X-ray spectrometry elemental maps of C and N, repectively. Scale bars; a , b (200 nm); d (5 nm); e , f , g (200 nm). Full size image Nitrogen sorption experiments were performed to examine the pore characteristics of the ZIF-8 precursor and the high-level N-doped graphene analogous particles ( Supplementary Figs 12–15 ; Supplementary Discussion ). In this study, the pore size of approximately 2 nm ( Supplementary Table 1 ) was larger than that of the nanoporous carbon (approximately 1 nm) that was obtained by direct carbonization of a commercially available ZIF-8 without any additional carbon sources [41] . On the basis of previous studies, a pore size of 2–10 nm facilitates rapid electrolyte transfer because the nanopores and interconnections provide more favourable pathways for ion penetration and transport [42] . Therefore, the as-prepared N-doped graphene analogous particles are suggested to be an excellent anode material for LIBs. The elemental analysis indicated that the N content decreased drastically as the pyrolysis temperature increased. The N-C-600 contained 25.99 wt% nitrogen (higher than that of previously reported N-doped carbon materials). However, not all of the N atoms were incorporated into the graphitic lattice because a high N-doped content can result in structural instability. Some N atoms existed as C≡N groups in the resulting N-doped graphene analogous particles, as revealed by Fourier transform infrared spectroscopy (FTIR) and TGA–IR–MS. As the pyrolysis temperature increased to 700, 800 and 900 °C, the N content decreased to 24.45, 17.72 and 10.73 wt%, respectively. More details regarding the as-prepared N-doped graphene analogous particles are summarized in Supplementary Table 2 . A large number of polyvinylpyrrolidone molecules adsorbed by the ZIF-8 framework could also serve as N and C sources in the final product ( Supplementary Note 3 ). To the best of our knowledge, the N content in the N-C-800 carbon materials is as high as 17.72 wt%, and is much greater than the N content reported in other N-doped carbon materials for LIBs (approximately 10 wt%). For example, Huang and colleagues [43] synthesized N-doped CNFWs with a N content of 10.25 wt% through the chemical activation of homemade Ppy nanofibre webs and KOH. The X-ray photoelectron spectroscopy (XPS) spectra ( Fig. 4 ) for N-C-700, N-C-800 and N-C-900 show that the N 1s spectrum can be deconvoluted into three peaks, pyridinic N (N-6, 398.4±0.2), pyrrolic or pyridonic N (N-5, 399.8±0.2) and quaternary N (400.7±0.4). N-5 represents pyrrolic N in a five-membered ring and contributes two electrons to the π system. N-6 is pyridinic N because the N atom substitutes a carbon atom in the C 6 ring and bonds with two sp 2 carbon atoms. N-Q is graphitic N, which is located inside the graphitic carbon plane and bonds with three sp 2 carbon atoms [44] , [45] . Supplementary Table 2 summarizes the fitting results for the N 1s spectra of the as-prepared N-doped graphene analogous particles. The N-5 and N-6 species are the dominant N-containing functional groups in all of the MOF-derived N-doped graphene analogous particles. The N-Q content increases as the carbonation temperature increases. The plentiful N-containing species (especially, N-5 and N-6) (ref. 46 ) serves as an electrochemically active site for enhancing the capacitive properties of the N-doped graphene analogous particles for the LIBs. Particularly, in N-C-700 and N-C-800, the N-6 content represents 50.38 and 43.21% of the total N, respectively, which is greater than in the N-CNFWs (approximately 36%) (ref. 37 ). Compared with the surface post modification (for example, the NH 3 treatment of porous carbon at high temperatures), our study provides a novel and facile method for producing N-doped graphene analogous particles. Furthermore, N-doped graphene analogous particles with different microstructure and N content can be conveniently generated by controlling the carbonization temperature of the MOF precursor. 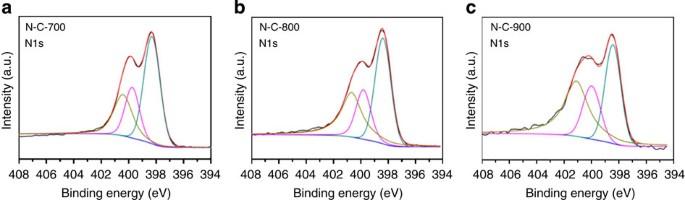Figure 4: N 1s spectra of N-doped graphene analogous particles obtained at different carbonization temperatures. (a) N-C-700, (b) N-C-800, and (c) N-C-900, respectively. Figure 4: N 1s spectra of N-doped graphene analogous particles obtained at different carbonization temperatures. ( a ) N-C-700, ( b ) N-C-800, and ( c ) N-C-900, respectively. Full size image The FTIR spectrum of the N-C-500 is similar to that of the ZIF-8 precursor ( Supplementary Fig. 16 ), which further demonstrates the high thermal stability of the ZIF-8 framework (as high as 500 °C). However, although the spectrum of each N-doped graphene particle analogues is complicated, the samples synthesized at different carbonization temperatures from 600 to 900 °C show a similar FTIR spectrum ( Fig. 5 ). The C=N bonding (approximately 1,600 cm −1 ) and N–H bonding (approximately 1,300 cm −1 ) forms of nitrogen are clearly observed. The band at 2,225 cm −1 is attributed to the nitrile C≡N groups [47] . Surprisingly, the intensity of the peak at 2,225 cm −1 decreases as the carbonation temperature increases. This band is almost invisible in N-C-800. The TGA–IR–MS results ( Supplementary Fig. 17 ) further show that the (CN) 2 molecules are released from N-C-600 and N-C-700. However, these molecules were not detected in the N-C-800, which demonstrated that no nitrile C≡N groups existed in the N-C-800. The pyridinic N and pyrrolic N in N-doped carbon materials are known to significantly contribute to Li storage. Therefore, it could be concluded that the partial N that exists as C≡N in the N-C-600 and N-C-700 samples is not beneficial for improving the specific capacity. Consequently, although the N content in N-C-700 is higher than that of N-C-800, the electrochemical performance of N-C-700 is not superior to that of N-C-800. In addition, as the carbonization temperature increases, the broad N–H peak at approximately 3,200 cm −1 in the N-rich carbon materials gradually weakens, indicating the gradual reduction of pyrrolic-type N in the N-doped graphene analogous particles [48] , which is consistent with the XPS analysis. 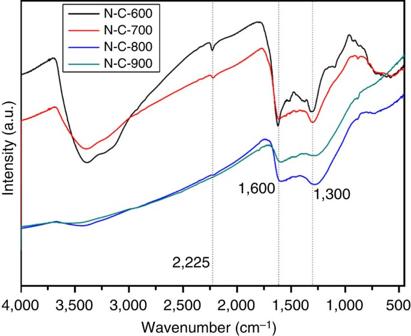Figure 5: IR spectra of N-doped graphene analogous particles obtained at different calcination temperatures. N-C-600, N-C-700, N-C-800, and N-C-900 stand for the samples prepared at 600, 700, 800, and 900 °C, respectively. Figure 5: IR spectra of N-doped graphene analogous particles obtained at different calcination temperatures. N-C-600, N-C-700, N-C-800, and N-C-900 stand for the samples prepared at 600, 700, 800, and 900 °C, respectively. Full size image Electrochemical performance as an anode material for LIBs The successful fabrication of high-level N-doped graphene analogous particles for a superior LIB anode is evident based on the excellent electrochemical performance of the LIBs. 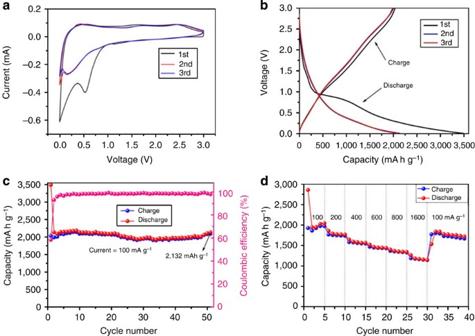Figure 6: Electrochemical performance of the N-C-800 electrode. (a) Cyclic voltammetry curve at 0.1 mV s−1scan rate. (b) Galvanostatic charge–discharge profiles at a current density of 100 mA g−1. The third curves exhibited significant overlap with the second charge and discharge curves. (c) Cycling performance at a current density of 100 mA g−1. (d) Rate performance at different current densities from 100 to 1,600 mA g−1. Figure 6a shows the first three cyclic voltammogram (CV) curves of the N-C-800 carbon electrode at room temperature between 0.0 and 3.0 V at a scan rate of 0.1 mV s −1 . Notably, the CV curve of the first cycle is different from the CV curves of the subsequent cycles, especially for the discharge brand. For the first discharge cycle, a strong peak is observed at 0.6 V, which is usually attributed to the occurrence of side reactions on the electrode surfaces and interfaces due to the solid-electrolyte interphase (SEI) film [45] . Moreover, the intensity of this peak during the first cycle is much stronger than the intensity during the following cycles, indicating the occurrence of some irreversible reactions and the formation of a SEI film. A distinct peak appears at 0.2 V during discharge from the second cycle onward, which could be ascribed to the generation of a new SEI film during the charge and discharge processes. From the second cycle onwards, it is important to note that the CV curves almost overlapped, indicating the stable and superior reversibility of the N-doped graphene analogous particles. Figure 6: Electrochemical performance of the N-C-800 electrode. ( a ) Cyclic voltammetry curve at 0.1 mV s −1 scan rate. ( b ) Galvanostatic charge–discharge profiles at a current density of 100 mA g −1 . The third curves exhibited significant overlap with the second charge and discharge curves. ( c ) Cycling performance at a current density of 100 mA g −1 . ( d ) Rate performance at different current densities from 100 to 1,600 mA g −1 . Full size image Figure 6b shows the discharge/charge profiles of the first three cycles for the N-doped graphene analogous particles at a current density of 100 mA g −1 between 0.01 and 3.0 V. The voltage profiles of the N-doped graphene analogous particles are similar to those previously reported for N-doped carbon materials [43] , [49] . The presence of a plateau at approximately 0.9 V in the first cycle can be ascribed to the formation of SEI films on the surfaces of the N-doped graphene analogous particles. The discharge curve in the first cycle is as high as 3,487 mAh g −1 , while its first reversible specific capacity is only 2,037 mAh g −1 , resulting in an initial coulombic efficiency of approximately 58.4%. This reversible specific capacity is much higher than that of the CNF derived from the polypyrrole web (1,280 mAh g −1 , 10.25% N) and the PMC-650 obtained from protein (approximately 1,780 mA h g −1 , 10.12% N) [43] , [49] . Wang and co-workers synthesized N-doped graphene with a N-doping level of 7.04 atom% by thermally annealing graphene and melamine. In this case, the reversible capacity was 1,136 mA h g −1 , when a relatively low current density of 50 mA g −1 was used [50] . Moreover, the relative low initial coulombic efficiency can be attributed to the irreversible capacity loss, including the formation of the SEI film and the decomposition of the electrolyte. These results also match the CV results in which the cathodic peaks are present in the first scan but absent in the following scans. However, the initial columbic efficiency was greater than the efficiency reported for the N-containing carbon materials, suggesting that the high-level N doping in the graphene analogous structure can reduce the extent of the irreversible capacity loss during the first cycle. These excellent performances could be attributed to the much higher N-doping levels (17.72 wt% N) in our materials. The cycling performance of the high-level N-doped graphene analogous particles was evaluated at 100 mA g −1 over a range of 0.01–3.0 V versus Li/Li + . As shown in Fig. 6c , the particles show excellent cyclic stability with a high capacity. After 50 cycles, the electrode still maintained a discharge capacity of 2,132 mA h g −1 , which is approximately 99.2% of the second electrode (2,150 mAh g −1 ). To the best of our knowledge, such an exceedingly high Li storage capacity has not been reported previously for an N-doped carbon-based anode material [43] , [49] , [50] . To understand the electrochemical performance of the as-prepared N-doped graphene analogous particles, we further studied the rate performance of an electrode. Figure 6d presents the rate capabilities and the cycle performance of an N-rich carbon electrode at various current densities (from 100 to 1,600 mA g −1 ). When the current density gradually increased from 100 to 200, 400, 600, 800 and 1,600 mA g −1 , the corresponding average discharge capacities decreased from 2,163, to 1,790, 1,588, 1,463, 1,361 and 1,182 mA h g −1 , respectively. If the current density became 100 mA g −1 again, the average discharge capacity returned to approximately 1,746 mA h g −1 , which indicated a very stable cycling performance. This result demonstrates that the MOF-derived N-doped graphene analogous particles (N-C-800) have a great potential as a high-rate anode material for LIBs. The electrochemical performance at a large current density of 500 mA g −1 across a voltage range of 0.01–3.0 V was evaluated for N-C-800 ( Supplementary Fig. 18 ). The reversible capacity is 1,123 mAh g −1 in the first cycle and retains 1,147 mAh g −1 after 200 cycles, which suggests an extraordinary electrochemical performance. In addition, the initial coulombic efficiency is 53.4%, which is higher than the other N-doped carbon-based materials. However, the coulombic efficiency increases dramatically on cycling, reaching over 98% after seven cycles and over 99.4% after 200 cycles. In general, larger current densities can destroy the structure of electrode materials and result in a rapid capacity loss [51] , [52] . However, as shown in Fig. 7 , an electrode prepared from N-C-800 maintained a capacity of 785 mAh g −1 after 1,000 cycles at 5 A g −1 . This result further demonstrates the excellent long-term cycling stability of the anode. 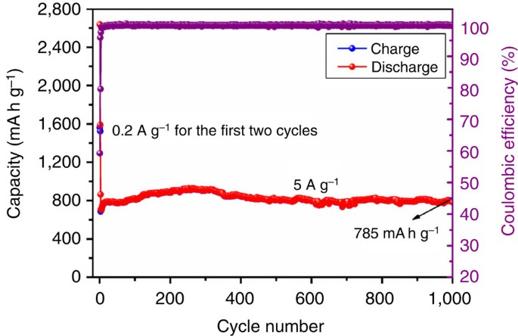Figure 7: Cycling performance of N-C-800 at a current density of 5 A g−1. To activate the electrode, a current density of 0.2 A g−1was used for the first two cycles, and then the cycling performance of the N-rich carbon materials was evaluated at 5 A g−1in the range of 0.01–3.0 V versus Li/Li+. Charge and discharge capacity curves are almost overlapping. Figure 7: Cycling performance of N-C-800 at a current density of 5 A g −1 . To activate the electrode, a current density of 0.2 A g −1 was used for the first two cycles, and then the cycling performance of the N-rich carbon materials was evaluated at 5 A g −1 in the range of 0.01–3.0 V versus Li/Li + . Charge and discharge capacity curves are almost overlapping. Full size image High-rate discharge and charging processes are important for many practical battery applications [53] , [54] , [55] , [56] , including their use in electric vehicles and portable power tools. The very high capacity, excellent cyclic performance and rate capabilities of the MOF-derived N-doped graphene analogous particles (N-C-800) make them a promising candidate as anode materials for high-performance LIBs. To the best of our knowledge, the N-C-800 shows a higher N content and better Li storage performance than reported for other N-doped carbon materials ( Supplementary Table 3 ). Furthermore, N-C-800 showed a superior Li storage performance as an anode material for LIBs in terms of high current densities ( Supplementary Table 4 ) and long-life cycles ( Supplementary Table 5 ). Notably, a long cycle life of more than 1,000 cycles is rarely reported in anode materials for LIBs. Such an enhanced electrochemical performance can be ascribed to the unique nanostructure of the N-C-800. Our N-doped carbon material can be considered as aggregates of small graphene analogous particles with N doping in the graphene honeycomb lattice and as modifications at the lattice edges. The aggregation of the small graphene analogous particles with the N atoms localized at their edges can generate large amounts of nanopores with their inner surfaces decorated with pyridinic and pyrrolic N, providing more active sites for Li storage and facilitating the transfer of Li ions and electrons in the electrode ( Fig. 8 ). Thus, the resulting sample shows a higher reversible capacity as an anode material for LIBs than normal N-doped graphene. The divacancy and Stone–Wales defects inevitably exist in the resulting N-doped graphene analogous particles [57] , [58] and would be beneficial for the adsorption of Li atoms according to previous reports [59] , [60] . However, graphene (approximately 568 mA h g −1 ) (ref. 13 ) and N-doped graphene (900 mA h g −1 ) (ref. 14 ) both contain divacancy and Stone–Wales defects and exhibited relatively lower capacities for Li storage relative to our samples, which suggests that the divacancy and Stone–Wales defects may contribute to, but not cause, the extra experimentally observed capacity. 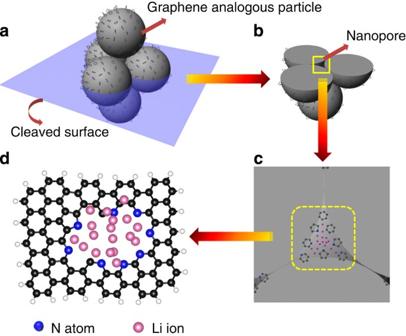Figure 8: Schematic representation of extra Li storage in N-doped graphene analogous particles. (a) The aggregate of the small graphene analogous particles with N atoms localized at their edges can generate large amounts of nanopores with their inner surface decorated with pyridinic and pyrrolic N, which also provide an extra capacity. (b) The cleaved surface of the aggregate. (c) The enlargement of a nanopore between the N-doped graphene analogous particles. (d) The theoretical calculations model of space for Li storage based on a graphene sheet with a hole containing eight N atoms at the edge. Figure 8: Schematic representation of extra Li storage in N-doped graphene analogous particles. ( a ) The aggregate of the small graphene analogous particles with N atoms localized at their edges can generate large amounts of nanopores with their inner surface decorated with pyridinic and pyrrolic N, which also provide an extra capacity. ( b ) The cleaved surface of the aggregate. ( c ) The enlargement of a nanopore between the N-doped graphene analogous particles. ( d ) The theoretical calculations model of space for Li storage based on a graphene sheet with a hole containing eight N atoms at the edge. 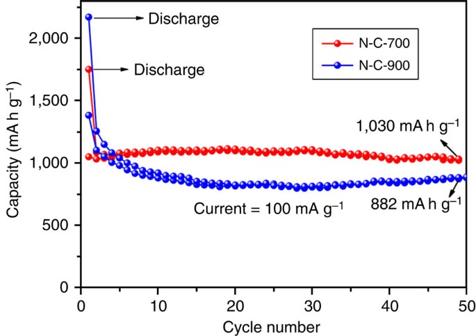Figure 9: Galvanostatic charge–discharge profiles of the N-C-700 and N-C-900 electrode at a current density of 100 mA g−1, respectively. To highlight the superiority of N-C-800 for anode materials for LIBs, the cycling performance of N-C-700 and N-C-900 was also investigated. Full size image Figure 9 shows the reversible charge/discharge capacity versus the cycle numbers of N-C-700 and N-C-900 at a current density of 100 mA g −1 between 0.01 and 3.0 V. The N-C-700 presents a better cycling stability and higher specific capacities than the N-C-900. The reversible capacities of the N-C-700 were 1,049 mAh g −1 in the first cycle and 1,030 mAh g −1 after 49 cycles. However, the reversible capacities of the N-C-900 were 1,381 mA h g −1 during the first cycle and 882 mA h g −1 after 49 cycles. Compared with the N-C-700, the curve for N-C-900 is not stable and the capacity decreases dramatically, which potentially results from its lower N content relative to N-C-700. In addition, the rate capabilities and cycle performances of N-C-700 and N-C-900 were investigated ( Supplementary Fig. 19 ). Figure 9: Galvanostatic charge–discharge profiles of the N-C-700 and N-C-900 electrode at a current density of 100 mA g −1 , respectively. To highlight the superiority of N-C-800 for anode materials for LIBs, the cycling performance of N-C-700 and N-C-900 was also investigated. Full size image In this case, the N-C-700 showed a better electrochemical performance than the N-C-900. However, the N-C-800 is the best anode material candidate for LIBs (relative to the N-C-700 and N-C-900) due to its high N doping in the analogous graphene structures, especially N-6. Although the N-C-700 has a greater N content than the N-C-800, the electrochemical performance of N-C-700 is poorer than that of N-C-800. This difference can be attributed to the temperature (700 °C), which is not optimal for the direct carbonization of ZIF-8. In this case, some N atoms exist as C≡N groups in N-C-700 (based on the IR and TGA–IR–MS results), which is not beneficial for Li storage. The N-C-900, which was obtained at a higher temperature, also showed a lower capacity than that of the N-C-800. Higher carbonation temperatures facilitate the formation of quaternary N based on the XPS results (44.26, 35.53 and 27.23 atom% for N-C-900, N-C-800 and N-C-700, respectively). Thus, the high quaternary N content in the lattice can increase the energy of the carbon framework. The structured instability would increase after undergoing many charge–discharge cycles. Hence, it is suggested that the high quaternary N content in N-C-900 results in the bad cycling performance [23] . To further investigate the outstanding electrochemical performance of N-C-800, TEM and SEM analysis were used to observe the morphology changes of the electrode after 20 charge/discharge cycles at 100 mA g −1 . From Supplementary Fig. 20 , it is obvious that the composite anode maintains its original appearance even after the long-term charge and discharge processes. In addition, the polyhedron-like aggregates of the N-doped graphene analogous particles are uniformly distributed in the composites of acetylene black and polyvinylidene fluoride (PVDF), further confirming that the unique structure can effectively alleviate the pulverization and prevent particle aggregation, ensuring the long-cycle stability. To better understand the N-doped graphene analogous particles, we performed density functional theory calculations using the Vienna Ab Initio Simulation Package [61] . The calculation details are described in the Supplementary Discussion . The density functional theory was calculated by Vienna Ab Initio Simulation Package using the supplied Projector Augmented Wave potentials for core electrons [62] . The N-C-800 can be considered as aggregates of multiple small graphene analogous particles based on the HRTEM and Raman characterization. Therefore, based on a single graphene analogous particle, we optimized the calculation model and constructed a single-layer graphene model to understand the edge N doping and electrochemical properties of the material. As a simplified model of the multilayer graphene cluster, a single-layer graphene cluster composed of 134 atoms (C 106 H 28 ) was examined and is illustrated in Supplementary Fig. 21 . The pristine graphene cluster is approximately 15 × 20 Å in size with all of the carbon atoms on the edges terminated with hydrogen atoms. The cluster consists of zigzag edges and armchair edges, which are the most common edge shapes of graphene without considering reconstruction [63] , [64] , [65] . A periodic boundary condition is used by adding vacuum space, and the separation between neighbouring clusters is not less than 15 Å in all three dimensions. We calculated the possible structure of high-level N-doped graphene analogous particles and the adsorption ability of the edge-doped graphene. The calculation results show that the edge-doped model is a favourable structure ( Supplementary Fig. 22 ) that can provide an extra capacity of 395.21 mAh g −1 ( Supplementary Figs 23–25 ; Supplementary Table 6 ). As discussed above, the N-C-800 can be considered as an aggregate of small graphene analogous particles. The aggregation of small graphene analogous particles with N atoms localized at their edges can generate large amounts of nanopores in their inner surfaces that are decorated with pyridinic and pyrrolic N. These nanopores may also provide extra capacity ( Fig. 8 ). To understand the Li storage in the nanopores qualitatively (space for Li storage), we conducted a theoretical study based on a simplified model with a large hole inside a 2D graphene sheet, as shown in Fig. 10a . The 2D graphene sheet with a large hole can be considered as the cleaved surface of an aggregate of the edge N-doped graphene analogous particles. Therefore, as shown in Fig. 8 , the hole represents a nanopore between the graphene analogous particles. The 2D cleaved surface is used instead of a 3D nanopore due to the difficulty of modelling and calculating the Li storage in a 3D nanopore. 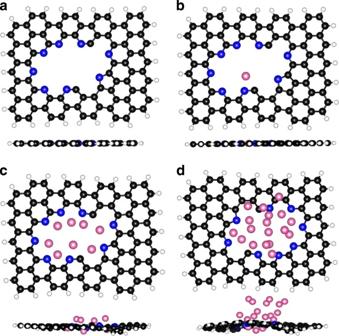Figure 10: A theoretical study on the Li storage in the nanopores with their inner surfaces decorated with pyridinic and pyrrolic N. (a) The simplified model with a large hole inside the 2D graphene and (b–d) the space for Li storage model with one, eight and eighteen Li atoms, respectively. (both from top view and side view) The black, blue, white and pink balls refer to carbon, nitrogen, hydrogen and lithium atoms, respectively. Figure 10: A theoretical study on the Li storage in the nanopores with their inner surfaces decorated with pyridinic and pyrrolic N. ( a ) The simplified model with a large hole inside the 2D graphene and ( b – d ) the space for Li storage model with one, eight and eighteen Li atoms, respectively. (both from top view and side view) The black, blue, white and pink balls refer to carbon, nitrogen, hydrogen and lithium atoms, respectively. Full size image The hole inside the graphene is large (10.2 Å in length and 6.0 Å in width), and is comparable in size to the N-C-800 nanopores. The pyrrolic N and pyridinic N doped at the edges of the large hole represent the N decoration on the inner surfaces of the nanopores. Therefore, the Li storage in the hole is very similar to the storage in an aggregate nanopore. However, although this model is a simplified structure, it is reasonable to study the Li storage mechanism qualitatively in space. We calculated the average potential of Li intercalation in the hole by using equation (3) (shown in the Supplementary Discussion ). To reduce the computation cost, we did not add the Li atoms one by one. Instead, we established and calculated nine models in which the Li atoms increased from one to 18. Some of the optimized structures are shown in Fig. 10b–d , and the average potential of Li intercalation for Li storage space is illustrated in Supplementary Fig. 26 . The average Li intercalation potential remains positive (0.43 V) when the eighteenth Li atom is embedded in the hole, which indicates that the Li storage capacity of the hole is greater than 18. Interestingly, as calculated above, each pyrrolic N or pyridinic N can adsorb two Li atoms. Therefore, the hole containing eight N atoms at the edge should adsorb sixteen Li atoms. However, the Li storage capacity from the eight N atoms at the edge was better than the Li storage capacity when the eight edge N atoms were separated in the model ( Supplementary Fig. 22a ), which should be described by the mechanism of Li storage. On the basis of the calculation results, we assumed that the origin of the space for Li storage could be the unsaturated nitrogen at the edge. That is, one pyrrolic N or pyridinic N cannot adsorb three Li atoms, while two Li atoms cannot saturate the adsorption ability of the N atom completely. Therefore, the pyridinic and pyrrolic N on the inner surface of a nanopore will function as a whole to adsorb more than sixteen Li atoms. Consequently, the Li storage in the nanopores and at the edge-doped N atoms of the graphene analogous particles can generate extra Li storage capacity, which is higher than 395.21 mAh g −1 . In summary, a high N content in graphene analogous particles contributes to a high specific capacity for Li storage. Avoiding oxidization at the edges of graphene sheets was found to provide numerous active sites for grafting N atoms. High-level N-doped graphene analogous particles (N-C-800) have been successfully fabricated by a facile and scalable synthesis method through direct carbonation of the N-containing MOFs (ZIF-8). This method resulted in an N content of up to 17.72 wt%. Furthermore, the resulting unique structure contains a large number of small graphene analogous particles that provide abundant active sites for grafting the nitrogen heteroatoms, especially for the pyridinic N or pyrrolic N. The N-C-800 material exhibited a highly reversible specific capacity of 2,132 mAh g −1 at a current density of 100 mA g −1 after 50 cycles, and 785 mAh g −1 at a high current density of 5 A g −1 after 1,000 cycles. Compared with existing N-doped carbon materials for LIBs, our MOF-derived N-doped graphene analogous particles showed excellent electrochemical performance, demonstrating that they should be considered as potential candidates for anode materials for high-performance LIBs. In addition, our approach offers a pathway for realizing high-level N doping in the bulk lattice and at the edges of the graphene sheets for energy storage. Preparation of the zeolitic imidazolate framework, ZIF-8 All chemicals were of analytical grade and were used without any further purification. During the typical synthesis procedure, a methanolic solution (50 ml) of zinc nitrate (Zn(NO 3 ) 2 ·6H 2 O, 120.0 mg) was added dropwise to a methanolic solution (50 ml) of 2-methylimidazole (105.0 mg) and polyvinylpyrrolidone (K-30, 0.3 g) using a syringe. The entire reaction process was performed at room temperature with agitated stirring. After stirring for 20 min, the reaction was aged at room temperature without any interruption for 10 h. The resulting white precipitate was centrifuged and washed several times with methanol before drying in an oven at 60 °C. Preparation of the N-doped graphene analogous particles The N-doped graphene analogous particles were synthesized by direct carbonization of the as-prepared ZIF-8 under a flow of nitrogen gas at temperatures of 500 to 900 °C. Typically, the ground ZIF-8 was homogeneously dispersed in a ceramic boat before placing the ceramic into a tube furnace. After the sample was exposed to a flow of nitrogen (400 ml min −1 ) at room temperature for 30 min, the furnace was heated to the targeted carbonization temperature using a heating rate of 5 °C min −1 . Then, the resulting sample was extensively washed using a 35% concentration of HCl to remove the residual Zn component. Next, the sample was washed several times with deionized water and absolute ethanol before drying in an oven at 60 °C. On the basis of the TGA data, the ZIF-8 was annealed at 500, 600, 700, 800 and 900 °C for 8 h using a heating rate of 5 °C min −1 under a N 2 atmosphere to obtain the related samples (referred to hereinafter as N-C-500, N-C-600, N-C-700, N-C-800 and N-C-900, respectively). Material characterization The powder XRD patterns of the samples were recorded with an X-ray diffractometer (Japan Rigaku D/MAX-γA) using Cu-Kα radiation ( λ =1.54178 Å) over a 2 θ range of 10–70°. FESEM images were collected on a JEOL JSM-6700 M scanning electron microscope. TEM images were taken on a Hitachi H-800 transmission electron microscope using an accelerating voltage of 200 kV, and a HRTEM (JEOL-2011) was operated at an accelerating voltage of 200 kV. The specific surface area was evaluated at 77 K (Micromeritics ASAP 2020) using the Brunauer–Emmett–Teller method, while the pore volume and pore size were calculated according to the Barrett–Joyner–Halenda formula applied to the adsorption branch. TGA was carried out using a Shimadzu-50 thermoanalyser under flowing nitrogen and at a heating rate of 10 °C min −1 . XPS was performed on an ESCALAB 250 X-ray photoelectron spectrometer using Al Ka radiation. The FTIR spectrum was determined using a Magna-IR 750 spectrometer over a range of 500–4,000 cm −1 with a resolution of 4 cm −1 . Electrochemical measurements The electrochemical behaviour of the N-doped graphene analogous particles was examined using CR2032 coin-type cells with lithium serving as the counter electrode and the reference electrode. The working electrode was prepared by mixing 50% of the active materials, 35% of the polymer binder (PVDF) and 15% of the conductive material (acetylene black) in N -methyl-2-pyrrolidone ( Supplementary Methods ). In a single experiment, the total mass of the active material, PVDF, and acetylene black was 40.0 mg (20.0 mg of active materials) when preparing a film on the surface of a copper foil current collector. The mixture was subsequently bush coated on copper foil and then dried at 80 °C for 12 h. The electrolyte used in the cells was 1.00 M LiPF 6 in ethylene carbonate and diethyl carbonate (EC:DEC=1:1). Then, approximately 20 electrodes were fabricated due to the low specific weights of the active materials (the crucible contained some residual mixture). In addition, to investigate the electrochemical performance of N-C-800, the rate capability was examined using CR2025 coin-type cells. The cells were assembled in an argon-filled glovebox with moisture and oxygen content of less than 1 p.p.m. The CR2032 coin-type cells (MBraun Labmaster 130) and CR2025 coin-type cells were assembled in argon-filled gloveboxes (Mikrouna, Super (1220/750/900)). The electrode capacity was measured using the galvanostatic discharge-charge method and employing a battery test system (Neware CT-3008 W) with a voltage range between 0.01 and 3.0 V. How to cite this article : Zheng, F. et al . High lithium anodic performance of super-high nitrogen-doped porous carbon prepared from a metal-organic framework. Nat. Commun. 5:5261 doi: 10.1038/ncomms6261 (2014).